Postmitotic control of sensory area specification during neocortical development The mammalian neocortex is subdivided into cytoarchitectural areas with distinct connectivity, gene expression and neural functions. Areal identity is initially specified by rostrocaudal and mediolateral gene expression gradients in neuroepithelial and radial glial progenitors (the ‘protomap’). On further differentiation, distinct sets of gene expression gradients arise in intermediate progenitors and postmitotic neurons, and are necessary to implement areal specification. However, it is still unknown whether postmitotic gene expression gradients can determine areal identity independently of protomap gradients. Here we show, by cell type-restricted genetic loss- and gain-of-function, that high levels of postmitotic COUP-TFI ( Nr2f1 ) expression are necessary and sufficient for the development of sensory (caudal) areal identity. Our data indicate a crucial role for postmitotic patterning genes in areal specification and reveal an unexpected plasticity in this process, which may account for complex and evolutionarily novel structures characteristic of the mammalian neocortex. The mammalian cerebral cortex is tangentially divided into numerous distinct cytoarchitectural domains, called areas, each specialized to process specific motor, sensory or multimodal inputs from cognate thalamic nuclei [1] , [2] , [3] . Each area is radially subdivided into six neuronal layers (laminae) characterized by specific cell types, morphologies and connectivity. Some previous studies have reported that both areal and laminar fates are specified in neocortical progenitor cells and determined at their last mitosis [4] , [5] . However, areal commitment begins much earlier than laminar fate determination. The first rough regionalization of the neocortical field (‘protomap’) starts around E8.5 and relies mainly on the interplay between morphogens (FGFs, BMPs and WNTs) and transcription factors (Pax6, Emx2, COUP-TFI and Sp8), expressed in and around the cortical neuroepithelium [6] , [7] , [8] , [9] . Neocortical neurons are generated from E10.5, when neuroepithelial progenitors differentiate into radial glia cells (RGCs) that initiate neurogenesis [10] . At the beginning of neurogenesis, RGCs have already begun to acquire a particular areal identity, which is then refined and implemented in neurogenic intermediate progenitors and postmitotic neurons [11] . Overall, previous studies have suggested that areal identity is initially defined in mitotically active RGCs. Recent studies have nevertheless shown that early laminar specification of neocortical neurons can be reprogrammed postmitotically by overexpressing Fezf2 , a transcription factor promoting the specification of layer V subcerebral projection neurons [12] , [13] . In addition, genetic inactivation of postmitotic transcription factors, such as Bhlhb5 and Tbr1 , impairs neocortical arealization [14] , [15] ; however, Bhlhb5 mutants show minor areal impairments, whereas in Tbr1 mutants the topography of thalamocortical connectivity could not be assessed due to deficient innervation, despite a clear shift of areal markers. Hence, it remains unclear whether these genes just refine and/or maintain initial areal commitment of newborn neurons or rather provide further information specifying areal domains. Most importantly, it is still uncertain whether initial cell cycle-determined regional specification is definitive or can be reversed during postmitotic phases of corticogenesis. In the present study, we have genetically manipulated postmitotic expression of the nuclear receptor COUP-TFI (RefSeq: Nr2f1 ), an areal patterning gene with graded, high-caudal to low-rostral expression in both progenitors and postmitotic neurons of developing neocortex [16] , [17] . Previous studies have shown that genetic inactivation of COUP-TF1 disrupts neocortical layering and arealization [18] , [19] , [20] , [21] , [22] . However, it is still unknown whether COUP-TFI regulates areal fate in progenitors (as suggested for most areal patterning genes) and/or in postmitotic neurons. To discern between these possibilities, we first ablated COUP-TFI function solely in postmitotic cortical cells and observed a significant expansion of frontal/motor areas at the expense of sensory ones. This phenotype is strikingly similar to that previously described after inactivating COUP-TFI throughout neocortical progenitors and neurons [18] , [22] , and demonstrates that COUP-TFI activity in progenitors alone is not sufficient to specify sensory cortex identity. To go beyond this analysis, we also genetically reintroduced COUP-TFI in postmitotic cortical neurons of COUP-TFI- null brains and found that its postmitotic expression partially rescues the caudal shift of sensory areas and the altered thalamocortical targeting. Ectopic expression of COUP-TFI in neurons of rostral neocortex suggests that its postmitotic activity is sufficient to reprogramme frontal/motor (F/M) areas into sensory ones. Taken together, these data support an important role for postmitotic patterning genes in neocortical arealization. Postmitotic inactivation of COUP-TFI As previously described, COUP-TFI is expressed in both neocortical progenitors and neurons, and is maintained at postnatal stages of development ( Fig. 1a and Supplementary Fig. 1a ). To selectively inactivate COUP-TFI in postmitotic cortical cells, we crossed COUP-TFI floxed mice [18] with a transgenic mouse line expressing Cre recombinase under control of the Nex promoter, which is active mainly in newborn cortical neurons from E11.5 onwards [23] , [24] , [25] ( Fig. 1a and Supplementary Fig. 1b ). As expected, in COUP-TFIfl/fl NexCRE mice (from now on NexCKO s), COUP-TFI was inactivated in late Tuj1+ neurons and in Tbr1+ preplate cells during early corticogenesis ( Supplementary Fig. 1c ), and in the upper subventricular zone, intermediate zone (IZ) and cortical plate (CP) cells during subsequent stages ( Supplementary Fig. 1d,e ) [26] . Moreover, we observed neither altered COUP-TFI expression nor Cre transcript in dorsal thalamic nuclei of NexCKO s, which might affect thalamic cell maturation and/or thalamocortical connectivity ( Fig. 1a and Supplementary Fig. 1b ). 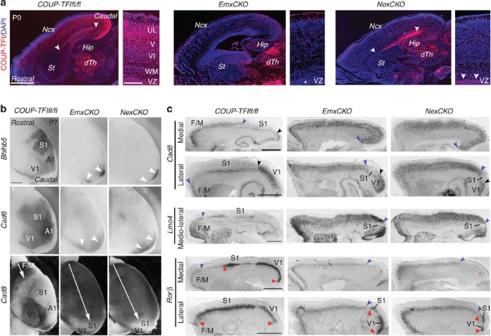Figure 1: Similar arealization defects inEmx-andNexCKOneocortices. (a) P0 brain sagittal sections from wt,Emx-andNexCKOmice immunolabelled for COUP-TFI. To the right of each sagittal section, high-magnification views of COUP-TFI expression along the radial extent of the somatosensory cortex. White arrowheads indicate the expression of COUP-TFI in the VZ. The asterisk indicates absence of COUP-TFI in the VZ of theEmxCKOs. In bothCKOs, COUP-TFI labels sparse cells in the cortex, which were previously shown to be interneurons migrating from the ventral telencephalon18,26. (b) Whole-mount P7 brains hybridized withBhlhb5andCad6(labelling sensory areas), andCad8(labelling mainly F/M and visual areas) riboprobes. BothCKObrains show reduced and caudalizedBhlhb5andCad6staining, and a corresponding expansion ofCad8expression. White arrowheads indicate sensory areas. White arrows indicate the expansion of F/M areas in bothEmx-andNexCKObrains. (c) Medial, mediolateral and lateral sagittal sections of P7 brains hybridized withCad8,Lmo4andRorβriboprobes, respectively. In bothCKObrains, the strong rostral expression ofCad8andLmo4is expanded caudally, whereas highRorβexpression domains are shifted to laterocaudal regions of the cortex. Blue arrowheads in sagittal sections hybridized withLmo4indicate the posterior boundary of highLmo4expression domains. Blue and black arrowheads delimit, respectively, anterior and posterior boundaries of a cortical domain corresponding to the primary somatosensory area (S1), in whichCad8is expressed at low levels in deep layers. Blue arrowheads in sagittal sections hybridized withRorßindicate caudal limits of a faintRorßexpression domain. Red arrowheads delimit cortical domains showing high levels ofRorßexpression (sensory areas). Red asterisks indicate the loss of cortical domains expressing high levels ofRorßinEmx-andNexCKOmedial sagittal sections. A1, primary auditory area; V1, primary visual area;Hip, hippocampus;dTh, dorsal thalamus; St, striatum. Scale bars, 200 μm (sagittal sections ina), 100 μm (cortical details ina), 900 μm (b), 600 μm (c). All panels of this figure are representative images of at least three independent experiments for each genotype. Figure 1: Similar arealization defects in Emx- and NexCKO neocortices. ( a ) P0 brain sagittal sections from wt, Emx- and NexCKO mice immunolabelled for COUP-TFI. To the right of each sagittal section, high-magnification views of COUP-TFI expression along the radial extent of the somatosensory cortex. White arrowheads indicate the expression of COUP-TFI in the VZ. The asterisk indicates absence of COUP-TFI in the VZ of the EmxCKOs . In both CKO s, COUP-TFI labels sparse cells in the cortex, which were previously shown to be interneurons migrating from the ventral telencephalon [18] , [26] . ( b ) Whole-mount P7 brains hybridized with Bhlhb5 and Cad6 (labelling sensory areas), and Cad8 (labelling mainly F/M and visual areas) riboprobes. Both CKO brains show reduced and caudalized Bhlhb5 and Cad6 staining, and a corresponding expansion of Cad8 expression. White arrowheads indicate sensory areas. White arrows indicate the expansion of F/M areas in both Emx- and NexCKO brains. ( c ) Medial, mediolateral and lateral sagittal sections of P7 brains hybridized with Cad8 , Lmo4 and Rorβ riboprobes, respectively. In both CKO brains, the strong rostral expression of Cad8 and Lmo4 is expanded caudally, whereas high Rorβ expression domains are shifted to laterocaudal regions of the cortex. Blue arrowheads in sagittal sections hybridized with Lmo4 indicate the posterior boundary of high Lmo4 expression domains. Blue and black arrowheads delimit, respectively, anterior and posterior boundaries of a cortical domain corresponding to the primary somatosensory area (S1), in which Cad8 is expressed at low levels in deep layers. Blue arrowheads in sagittal sections hybridized with Rorß indicate caudal limits of a faint Rorß expression domain. Red arrowheads delimit cortical domains showing high levels of Rorß expression (sensory areas). Red asterisks indicate the loss of cortical domains expressing high levels of Rorß in Emx- and NexCKO medial sagittal sections. A1, primary auditory area; V1, primary visual area; Hip , hippocampus; dTh , dorsal thalamus; St, striatum. Scale bars, 200 μm (sagittal sections in a ), 100 μm (cortical details in a ), 900 μm ( b ), 600 μm ( c ). All panels of this figure are representative images of at least three independent experiments for each genotype. Full size image To ensure that COUP-TFI was not altered in cycling progenitors of NexCKO cortices, we thoroughly investigated COUP-TFI expression in proliferating cells. First, we observed no changes in the number of double BrdU+/COUP-TFI+ cells between control ( COUP-TFIfl/fl ) and NexCKO neocortices ( Supplementary Fig. 1d and Supplementary Table 1 ). Likewise, we found no alterations in the total number of either cycling cells (Ki67+) or proliferating intermediate progenitors (Ki67+/Tbr2+) expressing COUP-TFI between the two conditions ( Supplementary Fig. 1e and Supplementary Table 1 ). Finally, the percentage of cells exiting (BrdU+/Ki67−) and re-entering the cell cycle (BrdU+/Ki67+) were unchanged between control and NexCKO cortices ( Supplementary Fig. 1f and Supplementary Table 1 ) differently from what was previously observed after inactivation of COUP-TFI in neuronal progenitors [19] . Taken together, these data indicate that COUP-TFI function is inactivated solely in cortical postmitotic cells of NexCKO brains. Postmitotic COUP-TFI inactivation severely affects areas To evaluate the role of postmitotically expressed COUP-TFI in neocortical areal specification, we compared arealization and lamination of NexCKO brains with those of COUP-TFIfl/fl EmxCre brains ( EmxCKO s), where COUP-TFI is inactivated in cortical precursors and neurons ( Fig. 1a ) [18] . Surprisingly, we observed a similar severe areal shift in both CKO s as compared with controls. In fact, the expression of Bhlhb5 , Cad6 and Rorß , which label sensory areas [15] , [27] , was reduced and shifted to the caudolateral rim of CKO neocortices ( Fig. 1b,c ), whereas normal rostral expression of Cad8 and Lmo4 (refs 27 , 28 ) (defining motor areas) expanded caudally ( Fig. 1b,c ). This indicates that presumed sensory areas (parietal cortex) abnormally express genes of rostral identity in the absence of COUP-TFI. Next, we investigated the laminar properties of motor and sensory areas, which are known to differ within the mammalian neocortex [29] . The laminar expression of Ctip2 in sensory areas is normally restricted to layer V subcerebral projection neurons [30] , whereas in both NexCKO and EmxCKO mutants it was abnormally upregulated in layers V and VI of the parietal cortex ( Fig. 2a,b and Supplementary Table 1 ), supporting motor-like respecification of presumed sensory regions [20] . Consistently, the number of cells coexpressing Ctip2 and layer VI markers, such as Tbr1, Fog2 (Gene: Zfpm2 ) and FoxP2 (refs 14 , 31 ), was increased in both CKO s compared with controls ( Supplementary Fig. 2a,b and Supplementary Table 1 ). We also observed some differences in the radial distribution of Tbr1-, Fog2- and Foxp2-positive cells between Nex- and EmxCKO s, indicating that COUP-TFI may promote, at least in part, the laminar specification of early-born neuronal populations in progenitor cells. In contrast, the expression of Bhlhb5 and Cux1 (refs 15 , 32 ) in upper layer neurons of the parietal cortex was lost in both CKO s, while their expression was maintained in occipital regions ( Supplementary Fig. 2c ). These data indicate a laminar mis-specification of COUP-TFI CKO primary somatosensory (S1) cortices, which tend to acquire layer-specific features of motor/frontal cortices. 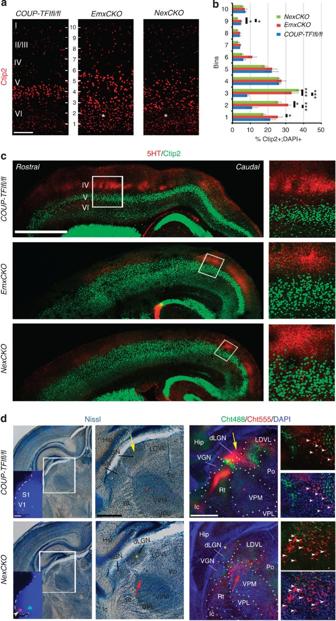Figure 2: Layering and innervation ofEmx-andNexCKObrains are affected. (a) Details of coronal sections from wt,Nex-andEmxCKOP7 somatosensory cortices immunolabelled for Ctip2. Asterisks indicate increased Ctip2 expression in layer VI ofCKOs.(b) Analysis of the radial distribution of Ctip2+ cells in parietal cortices (n=3 for each genotype) shows a significant increase in the number of these neurons in bins 2 (PANOVA<0.01) and 3 (PANOVA<0.005), corresponding to layer VI of bothCKOs. Detailed statistical data are listed inSupplementary Table 1. (c) Lateral sagittal sections from P7 brains immunolabelled with serotonin (5HT) and Ctip2. To the right, high-magnification views of the boxes depicted in left panels. (d) Coronal sections of P7 brains injected with CTB-conjugated fluorophores, Cht488 (green) and Cht555 (red), in medial and lateral regions of the occipital cortex (insets in left panel column) (n=3 for each genotype). Adjacent sections were stained with Nissl (white boxes indicate the regions magnified to the right) and DAPI (right panels). In controls, both dyes label the V1-related thalamic dorsal lateral geniculate nucleus (dLGN, yellow arrows) but not the ventral posteromedial nucleus (VPM, red asterisks), which sends axons to S1. InNexCKOs, the VPM is labelled by Cht555 (red arrow), in line with altered sensory areal positioning (yellow arrowhead in left panels insets). The dotted lines define thalamic nuclei in DAPI-stained sections. To the right, high magnification views of dLGN (yellow arrows) and VPM (red arrows) in controls andNexCKOsections, respectively. White arrowheads indicate labelled cell nuclei. Hip, hippocampus; ic, internal capsule; LDVL, laterodorsal thalamic nuclei; Po, posterior nucleus; Rt, reticular nucleus; VGN, ventral geniculate nucleus; VPL, ventral posterolateral nuclei; scale bar, 200 μm (a), 900 μm (cand left panels ofd), 300 μm (medial panels ind), 150 μm (right square panels ind). Statistical data from wt,Emx-andNexCKOwere compared by analysis of variance (ANOVA).Post-hocanalysis was performed by two-tailedt-test. *P-value ≤0.05, ***P-value ≤0.005 (two-tailedt-test),n=3. Error bars represent s.e.m. Figure 2: Layering and innervation of Emx- and NexCKO brains are affected. ( a ) Details of coronal sections from wt, Nex- and EmxCKO P7 somatosensory cortices immunolabelled for Ctip2. Asterisks indicate increased Ctip2 expression in layer VI of CKOs. ( b ) Analysis of the radial distribution of Ctip2+ cells in parietal cortices ( n= 3 for each genotype) shows a significant increase in the number of these neurons in bins 2 ( P ANOVA <0.01) and 3 ( P ANOVA <0.005), corresponding to layer VI of both CKOs . Detailed statistical data are listed in Supplementary Table 1 . ( c ) Lateral sagittal sections from P7 brains immunolabelled with serotonin (5HT) and Ctip2. To the right, high-magnification views of the boxes depicted in left panels. ( d ) Coronal sections of P7 brains injected with CTB-conjugated fluorophores, Cht488 ( green ) and Cht555 ( red ), in medial and lateral regions of the occipital cortex (insets in left panel column) ( n =3 for each genotype). Adjacent sections were stained with Nissl (white boxes indicate the regions magnified to the right) and DAPI (right panels). In controls, both dyes label the V1-related thalamic dorsal lateral geniculate nucleus (dLGN, yellow arrows) but not the ventral posteromedial nucleus (VPM, red asterisks), which sends axons to S1. In NexCKOs , the VPM is labelled by Cht555 (red arrow), in line with altered sensory areal positioning (yellow arrowhead in left panels insets). The dotted lines define thalamic nuclei in DAPI-stained sections. To the right, high magnification views of dLGN (yellow arrows) and VPM (red arrows) in controls and NexCKO sections, respectively. White arrowheads indicate labelled cell nuclei. Hip, hippocampus; ic, internal capsule; LDVL, laterodorsal thalamic nuclei; Po, posterior nucleus; Rt, reticular nucleus; VGN, ventral geniculate nucleus; VPL, ventral posterolateral nuclei; scale bar, 200 μm ( a ), 900 μm ( c and left panels of d ), 300 μm (medial panels in d ), 150 μm (right square panels in d ). Statistical data from wt, Emx- and NexCKO were compared by analysis of variance (ANOVA). Post-hoc analysis was performed by two-tailed t -test. * P -value ≤0.05, *** P -value ≤0.005 (two-tailed t -test), n =3. Error bars represent s.e.m. Full size image To further compare areal specification in both CKO s, we investigated the topography of thalamocortical innervation, a major identifying feature of neocortical areas. An initial molecular analysis suggested impaired thalamocortical connectivity in both Nex- and EmxCKO cortices. First, in both CKO s we observed similar caudal expansion of Igfbp4 expression, which is normally excluded from territories receiving geniculocortical innervation (that is, primary visual area, or V1) [33] ( Supplementary Fig. 3a ). Second, subplate (SP) cells, which play an important role in conferring positional information to incoming thalamocortical axons (TCAs) [34] , [35] , appeared abnormally specified in both Nex- and EmxCKO s ( Supplementary Fig. 3b ). The normal high-rostral to low-caudal expression gradient of Ctgf , a well-known SP cell marker [36] , was inverted and slightly shifted to caudolateral neocortical territories in CKO brains. Notably, although Ctgf expression strongly decreased in both Nex- and EmxCKO s, its levels were inversely correlated to COUP-TFI dosage in neocortical progenitors ( Supplementary Fig. 3b ). This indicates that SP cell specification might rely both on mitotic and postmitotic COUP-TFI function. Finally, RORß expression, which regulates barrel formation on innervation of layer IV neurons by TCA [37] ( Fig. 1c ), and serotonin, a neurotransmitter labelling TCAs in primary sensory areas, were strongly caudalized in both CKO s ( Fig. 2c ). These data support the previously described caudalization of sensory TCAs in EmxCKO s [18] and envisage a similar connectivity defect in NexCKO brains. Accordingly, the injection of cholera toxin β-subunit (CTB)-conjugated fluorophores in the occipital postnatal cortex retrogradely labelled neurons of the dorsal lateral geniculate nucleus (dLGN) in controls and, in contrast, labelled neurons of the ventral posteromedial nucleus (VPM, normally connected to S1) in NexCKO s ( Fig. 2d ). Overall, comparison between Nex- and EmxCKO mutants revealed that postmitotic function of COUP-TFI is necessary for correct areal and laminar specification of neocortical neurons. Reduction of caudal enriched genes in NexCKO cortical neurons To obtain an overall picture of the molecular mechanisms underlying COUP-TFI function in postmitotic cells, we used Affymetrix arrays to profile changes of gene expression in mid-gestation neocortices of NexCKOs compared with littermate controls ( Fig. 3a and Supplementary Fig. 4 ). Among the top 20 genes up- or downregulated in mutant cortices (first screened for P -value <0.01 to select the most significant results) ( Supplementary Table 2 ), several genes were previously shown to be markers of rostral or caudal identity in the embryonic cortex [14] , [38] , suggesting that rostrocaudal identity was perturbed. This was confirmed by gene set analysis by using previously defined gene sets that represent rostral or caudal identity in specific cortical differentiation zones [38] . Overall, caudal-enriched genes were quantitatively reduced in the CP, SP and IZ cells of COUP-TFI mutants ( Fig. 3a and Supplementary Fig. 4a ). Examples of caudal marker genes with reduced expression included Cck , Chrna7 and Nefm in the CP; Cdh11 and Ngfr in the SP; and Bhlhb5 in the IZ. Interestingly, one caudal CP marker, Crabp1 , was significantly up- rather than downregulated in COUP-TFI mutant neocortices. This is consistent with previous studies showing that Crabp1 is directly repressed by COUP-TFI [39] and suggests that COUP-TFI may promote and limit caudal rather than inhibit rostral differentiation of postmitotic neurons during corticogenesis ( Fig. 3c ). 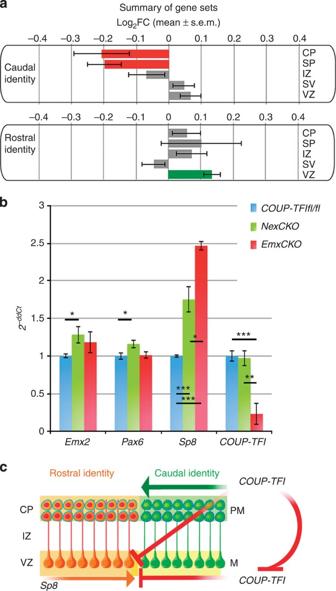Figure 3: Gene set and quantitative analyses of genes differentially expressed inNexCKObrains. (a) Summaries of the gene set analysis performed on genes differentially expressed between E15.5NexCKOand control neocortices. Significant changes (P-value <0.05, one-tailedt-test) with mean log2FC>0.1 are coloured green for increased intensity or red for decreased intensity. The data highlight that expression of caudal genes is significantly decreased in the CP and SP, whereas a few rostral genes are significantly increased in the VZ and, to a lesser extent, in postmitotic cells. See alsoSupplementary Fig. 3andSupplementary Table 2. (b) Graph plot of the fold enrichment of mitotic patterning genes from quantitative PCR analysis performed onRNAextracted from control,Nex-andEmxCKOE12.5 neocortices. The plot shows a mild but significant increase inPax6andEmx2expression only inNexCKObrains compared with controls (PPax6=0.05;PEmx2<0.05,n=3, two-tailedt-test). It also indicates a progressive increase ofSp8expression fromNex-toEmxCKObrains (PANOVA<0.001,n=3,post-hocanalysis: two-tailedt-test).COUP-TFIexpression levels inNexCKOsare not significantly different from control ones (P=0.875), despite its absence in postmitotic cells, whereas inEmxCKO, COUP-TFItranscript levels are strongly decreased when compared with both control andNexCKOsamples (PANOVA<0.01). (c) Hypothetical model representing the function of mitotically (m) and postmitotically (pm) expressed COUP-TFI. Although mitotic COUP-TFI has a role in the inhibition ofSp8expression, postmitotic COUP-TFI directly promotes caudal fate in neurons and indirectly downregulates mitoticCOUP-TFIandSp8expression. CP, cortical plate; IZ, intermediate zone; VZ, ventricular zone. All statistical data are detailed inSupplementary Table 1. Statistical data from wt,Emx-andNexCKOwere compared using the analysis of variance (ANOVA).Post-hocanalysis was performed by two-tailedt-test analysis. *P-value ≤0.05; **P-value ≤0.01; ***P-value ≤0.005 (two-tailedt-test),n=3 for each genotype. Error bars represent s.e.m. Figure 3: Gene set and quantitative analyses of genes differentially expressed in NexCKO brains. ( a ) Summaries of the gene set analysis performed on genes differentially expressed between E15.5 NexCKO and control neocortices. Significant changes ( P -value <0.05, one-tailed t -test) with mean log 2 FC>0.1 are coloured green for increased intensity or red for decreased intensity. The data highlight that expression of caudal genes is significantly decreased in the CP and SP, whereas a few rostral genes are significantly increased in the VZ and, to a lesser extent, in postmitotic cells. See also Supplementary Fig. 3 and Supplementary Table 2 . ( b ) Graph plot of the fold enrichment of mitotic patterning genes from quantitative PCR analysis performed on RNA extracted from control, Nex- and EmxCKO E12.5 neocortices. The plot shows a mild but significant increase in Pax6 and Emx2 expression only in NexCKO brains compared with controls ( P Pax6 =0.05; P Emx2 <0.05, n =3, two-tailed t -test). It also indicates a progressive increase of Sp8 expression from Nex- to EmxCKO brains ( P ANOVA <0.001, n =3, post-hoc analysis: two-tailed t -test). COUP-TFI expression levels in NexCKOs are not significantly different from control ones ( P =0.875), despite its absence in postmitotic cells, whereas in EmxCKO, COUP-TFI transcript levels are strongly decreased when compared with both control and NexCKO samples ( P ANOVA <0.01). ( c ) Hypothetical model representing the function of mitotically (m) and postmitotically (pm) expressed COUP-TFI. Although mitotic COUP-TFI has a role in the inhibition of Sp8 expression, postmitotic COUP-TFI directly promotes caudal fate in neurons and indirectly downregulates mitotic COUP-TFI and Sp8 expression. CP, cortical plate; IZ, intermediate zone; VZ, ventricular zone. All statistical data are detailed in Supplementary Table 1 . Statistical data from wt, Emx- and NexCKO were compared using the analysis of variance (ANOVA). Post-hoc analysis was performed by two-tailed t -test analysis. * P -value ≤0.05; ** P -value ≤0.01; *** P- value ≤0.005 (two-tailed t -test), n =3 for each genotype. Error bars represent s.e.m. Full size image Postmitotic COUP-TFI function inhibits rostral mitotic genes Genomic analysis also showed that markers of rostral identity were mostly unaffected in COUP-TFI mutants, except for an overall moderate upregulation of rostral ventricular zone (VZ) transcripts ( Fig. 3a and Supplementary Fig. 4b ). As COUP-TFI expression in progenitors was not directly affected by NexCre -mediated recombination ( Supplementary Fig. 1d,e ), the upregulation of rostral VZ markers presumably represents an indirect feedback effect. To investigate whether this hypothetical feedback regulates the expression of mitotic areal patterning genes, we analysed transcript levels of Pax6 , Emx2 , Sp8 and COUP-TFI itself, at E12.5, a stage at which they are all strongly expressed in progenitor cells ( Fig. 3b ). Although Emx2 and Pax6 transcript levels were only slightly affected in NexCKO s, the expression of Sp8 , a gene promoting rostral (motor) identity [40] , [41] , [42] , progressively increased from Nex- to EmxCKO cortices, suggesting a double (mitotic and postmitotic) control of COUP-TFI on Sp8 expression ( Fig. 3b and Supplementary Table S1 ). We also found that expression of COUP-TFI, despite its loss in postmitotic cells ( Supplementary Fig. 1c ), was unchanged in E12.5 NexCKO brains compared with controls. This might suggest an increased expression of COUP-TFI at the mitotic level, which is normally downregulated by postmitotic COUP-TFI expression at early stages. Thus, our molecular data describe a complex scenario in which COUP-TFI postmitotic function not only promotes caudal-related gene expression in neurons but also selectively inhibits expression of rostral mitotic patterning genes ( Fig. 3c ). Postmitotic COUP-TFI overexpression rescues areal defects Once determined that postmitotic COUP-TFI activity is necessary for correct neocortical arealization, we investigated whether its postmitotic expression is also sufficient to promote caudal identity. To this aim, we adopted a complementary strategy with respect to NexCKOs , that is, reintroducing COUP-TFI expression in postmitotic cells of COUP-TFI- null ( KO ) cortices. We first crossed the CAGGS-lox-stop-lox-hCOUP-TFI mouse line [43] (from now on ind/hCOUP-TFI ), which conditionally expresses the human orthologue of COUP-TFI (98% similarity with the murine sequence [44] ) under the control of a ubiquitous promoter, with the NexCre line ( Supplementary Fig. 5a–c ). Next, by crossing this new line ( iz/hCOUP-TFI ) with COUP-TFI constitutive KO s, we obtained COUP-TFI KO iz/hCOUP-TFI mice ( KO;iz/hCOUP-TFI ), which postmitotically overexpress hCOUP-TFI both in rostral and caudal regions of KO cortices ( Supplementary Fig. 5d ). Unfortunately, both constitutive KO [45] and KO;iz/hCOUP-TFI mice died at birth, limiting our analysis to P0 pups. To first validate the postmitotic to mitotic feedback model, we analysed mitotic patterning gene expression in E13.5 brains from loss- and gain-of-function embryos. In good accordance with the quantitative PCR analysis, we found no evident alterations either in the expression gradient or in the expression levels of Emx2 or Pax6 among wt, NexCKO and KO;iz/hCOUP-TFI brains ( Supplementary Fig. 6 ). However, Sp8 expression was respectively increased in NexCKO and strongly downregulated in KO;iz/hCOUP-TFI compared with wt brains ( Supplementary Fig. 6 ). These data support the model of a selective negative feedback exerted by postmitotic COUP-TFI on the expression of specific mitotic rostralizing factors ( Fig. 3c ). Next, we compared regionalized gene expression in loss- and gain-of-function P0 brains to corroborate COUP-TFI postmitotic role in areal patterning. First, the strong decrease in Bhlhb5 and caudal shift of Cad8 and Id2 expression in upper layers of COUP-TFI KO s indicated, despite the presence of mitotic COUP-TFI expression in NexCKOs , a comparable expansion of rostral domains between NexCKO and KO brains ( Fig. 4a–c ). Second, overexpression of hCOUP-TFI in postmitotic neocortical neurons ( KO;iz/hCOUP-TFI brains) rescued Bhlhb5 , Cad8 and Id2 regionalized expression profiles in parietal and occipital neocortices ( Fig. 4a,b ). Third, the reintroduction of COUP-TFI in postmitotic cells also restored correct layer specification, which was altered in loss-of-function mutant brains. Normal laminar expression of Ctip2 in layer V and Rorß expression in layer IV, which were strongly impaired in both NexCKO and COUP-TFI KO brains, were recovered in the parietal cortex of KO;iz/hCOUP-TFI mice ( Fig. 4c–e , Supplementary Fig. 7a,b and Supplementary Table 1 ). Moreover, hCOUP-TFI overexpression remarkably restored proper Ctgf gradient, which was inverted in both NexCKO and COUP-TFI KO brains ( Supplementary Fig. 7c ). Notably, Ctgf expression levels decreased more in constitutive KO s, where COUP-TFI is absent in all cortical cells, suggesting that both mitotic and postmitotic COUP-TFI functions regulate Ctgf expression levels. 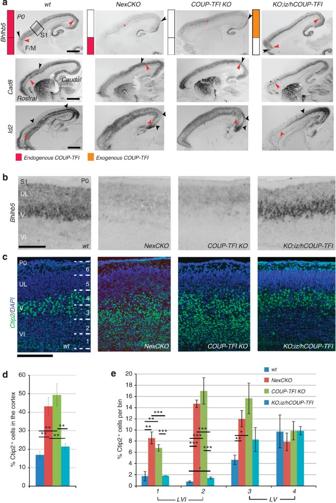Figure 4: Postmitotic rescue of areal and laminar defects. (a)In situhybridization withBhlhb5,Cad8andId2riboprobes on P0 sagittal sections fromwt,NexCKO,COUP-TFI KOandKO;iz/hCOUP-TFIbrains.Bhlhb5expression in upper layers (UL, black arrowheads) is caudalized, whereas in layer V its expression is lost (red asterisks) in bothNexCKOand constitutiveKObrains. InKO;iz/hCOUP-TFIbrains,Bhlhb5expression is rescued.Cad8expression in rostral UL (black arrowheads) and in layer V (red arrowheads) is caudally expanded in both loss-of-function mutants.KO;iz/hCOUP-TFIbrains show noCad8expression in UL (asterisk) and restored expression in parietal layer V (red arrowhead).Id2is normally expressed in rostral and caudal UL (black arrowheads), and in layer V of sensory areas (red arrowheads)27.hCOUP-TFIoverexpression (KO;iz/hCOUP-TFI)rescues normalId2expression in layer V of the parietal cortex (red arrowhead) and in caudal UL (black arrowhead), but not in rostral UL (black asterisk). (b) Details from P0 parietal cortices hybridized with showing restoredBhlhlb5expression inKO;iz/hCOUP-TFIbrains. (c) Details from coronal sections of P0 parietal cortices immunolabelled for Ctip2 showing restored Ctip2 expression in layer V ofKO;iz/hCOUP-TFIbrains. Numbers indicate the bins used inefor statistical analysis. (d) Plot depicting the different Ctip2+ cell percentages in the cortex of P0 brains from different conditions represented inc. (PANOVA<0.005). (e) Statistical analysis of Ctip2+ cells distribution showed a significant increase in Ctip2 expression in layers VI (bins 1, 2) and V (bins 3) of COUP-TFI mutants and its rescue inKO;iz/hCOUP-TFIbrains (bin 1:PANOVA<0.005; bin 2:PANOVA<0.005; bin 3:PANOVA<0.05;post hocanalysis: two tailedt-test). See alsoSupplementary Table 1. Scale bars, 200 μm (a), 50 μm (b,c). *P-value ≤0.05; **P-value ≤0.01; ***P-value ≤0.005 (two-tailedt-test),n=3 for each genotype. Error bars represent s.e.m. Figure 4: Postmitotic rescue of areal and laminar defects. ( a ) In situ hybridization with Bhlhb5 , Cad8 and Id2 riboprobes on P0 sagittal sections from wt , NexCKO , COUP-TFI KO and KO;iz/hCOUP-TFI brains. Bhlhb5 expression in upper layers (UL, black arrowheads) is caudalized, whereas in layer V its expression is lost (red asterisks) in both NexCKO and constitutive KO brains. In KO;iz/hCOUP-TFI brains, Bhlhb5 expression is rescued. Cad8 expression in rostral UL (black arrowheads) and in layer V (red arrowheads) is caudally expanded in both loss-of-function mutants. KO;iz/hCOUP-TFI brains show no Cad8 expression in UL (asterisk) and restored expression in parietal layer V (red arrowhead). Id2 is normally expressed in rostral and caudal UL (black arrowheads), and in layer V of sensory areas (red arrowheads) [27] . hCOUP-TFI overexpression ( KO;iz/hCOUP-TFI) rescues normal Id2 expression in layer V of the parietal cortex (red arrowhead) and in caudal UL (black arrowhead), but not in rostral UL (black asterisk). ( b ) Details from P0 parietal cortices hybridized with showing restored Bhlhlb5 expression in KO;iz/hCOUP-TFI brains. ( c ) Details from coronal sections of P0 parietal cortices immunolabelled for Ctip2 showing restored Ctip2 expression in layer V of KO;iz/hCOUP-TFI brains. Numbers indicate the bins used in e for statistical analysis. ( d ) Plot depicting the different Ctip2+ cell percentages in the cortex of P0 brains from different conditions represented in c . ( P ANOVA <0.005). ( e ) Statistical analysis of Ctip2+ cells distribution showed a significant increase in Ctip2 expression in layers VI (bins 1, 2) and V (bins 3) of COUP-TFI mutants and its rescue in KO;iz/hCOUP-TFI brains (bin 1: P ANOVA <0.005; bin 2: P ANOVA <0.005; bin 3: P ANOVA <0.05; post hoc analysis: two tailed t -test). See also Supplementary Table 1 . Scale bars, 200 μm ( a ), 50 μm ( b , c ). * P -value ≤0.05; ** P -value ≤0.01; *** P -value ≤0.005 (two-tailed t -test), n =3 for each genotype. Error bars represent s.e.m. Full size image Finally, we investigated whether the postmitotic re-expression of hCOUP-TFI significantly rescued the impairments in TCA topography, previously described in COUP-TFI KO brains [22] . Inserting lipophilic DiI and DiD crystals in medial and lateral regions, respectively, of the occipital cortex, we retrogradely labelled thalamocortical connections targeting presumed V1 area in the occipital cortex. As expected, both dyes labelled dLGN neurons in wild type (wt) and VPM neurons in the COUP-TFI KO , whereas both nuclei (dLGN and VPM) were retrogradely labelled in the KO;iz/hCOUP-TFI , indicating a partial rescue of visual thalamocortical connectivity ( Fig. 5 ). Thus, re-expression of hCOUP-TFI exclusively in postmitotic cells of COUP-TFI KO cortices can restore several area-specific features of sensory areas, such as regionalized gene expression, laminar cytoarchitecture and thalamocortical connectivity. 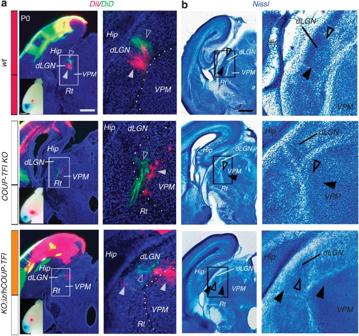Figure 5: Postmitotic rescue of thalamocortical topography. (a) Coronal sections from P0 brains (n=3 per genotype) in which DiI and DiD crystals (red and blue, respectively, in insets depicting whole-brain bright-field images, and red and green, respectively, in fluorescent images) were inserted in the occipital cortex. Inwtbrains, both lipophilic dyes retrogradely labelled cells of the dorsal lateral geniculate nucleus (dLGN), which sends axons to the primay visual area (V1), whereas inCOUP-TFI KOs both dyes labelled neurons in the ventral posteromedial nucleus (VPM), which is connected to the primary somatosensory area (S1). This shift in thalamocortical connectivity was partially rescued inKO;iz/hCOUP-TFIbrains, where DiD labelled neurons of the dLGN and DiI labelled neurons of both the dLGN and the VPM. White arrowheads and white empty arrowheads indicate cells retrogradely labeled by DiI and DiD, respectively. Right panels of each genotype represents higher magnifications of details depicted by squared boxes in left panels. (b) Brain coronal slices adjacent to those depicted inaand stained with Nissl. Right panels are higher magnifications of boxes depicted in left panels. Black and empty arrowheads represent, respectively, DiI and DiD labelled regions. Hip, hippocampus; Rt, reticular nucleus. Scale bars, 1 mm (whole brain bright-field images ina), 600 μm (coronal sections ina,b). All panels of this figure are representative images of at least three brains for each genotype. Figure 5: Postmitotic rescue of thalamocortical topography. ( a ) Coronal sections from P0 brains ( n =3 per genotype) in which DiI and DiD crystals (red and blue, respectively, in insets depicting whole-brain bright-field images, and red and green, respectively, in fluorescent images) were inserted in the occipital cortex. In wt brains, both lipophilic dyes retrogradely labelled cells of the dorsal lateral geniculate nucleus (dLGN), which sends axons to the primay visual area (V1), whereas in COUP-TFI KO s both dyes labelled neurons in the ventral posteromedial nucleus (VPM), which is connected to the primary somatosensory area (S1). This shift in thalamocortical connectivity was partially rescued in KO;iz/hCOUP-TFI brains, where DiD labelled neurons of the dLGN and DiI labelled neurons of both the dLGN and the VPM. White arrowheads and white empty arrowheads indicate cells retrogradely labeled by DiI and DiD, respectively. Right panels of each genotype represents higher magnifications of details depicted by squared boxes in left panels. ( b ) Brain coronal slices adjacent to those depicted in a and stained with Nissl. Right panels are higher magnifications of boxes depicted in left panels. Black and empty arrowheads represent, respectively, DiI and DiD labelled regions. Hip, hippocampus; Rt, reticular nucleus. Scale bars, 1 mm (whole brain bright-field images in a ), 600 μm (coronal sections in a , b ). All panels of this figure are representative images of at least three brains for each genotype. Full size image Ectopic COUP-TFI promotes caudal identity in rostral cortex The high ectopic expression of COUP-TFI in rostral cortex of KO;iz/hCOUP-TFI gave us the opportunity to test its function in a region normally characterized by low COUP-TFI expression ( Fig. 1a ). Although Lmo4 is normally expressed at high levels in upper layers of frontal and occipital (prospective visual) but not parietal cortical regions at P0, its expression was upregulated in the presumptive COUP-TFI KO S1, as observed by whole-mount in situ hybridization ( Fig. 6a ), sagittal sections ( Fig. 6b ) and immunolabelling ( Fig. 6c ). On the contrary, Bhlhb5 , which is normally highly expressed in S1 but not in F/M, was downregulated in S1 of COUP-TFI KO brains ( Fig. 6b,c ). High ectopic rostral expression of hCOUP-TFI was sufficient to downregulate Lmo4 and to upregulate Bhlhb5 expression ( Fig. 6b,c ) in F/M regions. Similarly, Cad8 , highly expressed in controls and COUP-TFI KO upper layers, was downregulated in F/M of KO;iz/hCOUP-TFI brains ( Fig. 6b ). As expression of these markers in F/M KO;iz/hCOUP-TFI cortices is reminiscent of their normal expression profiles in parietal/somatosensory cortex (S1 in Fig. 6b,c ), it is very likely to be that high rostral expression of hCOUP-TFI was sufficient to reprogramme motor/rostral to sensory/caudal identity. Interestingly, Lmo4 whole-mount in situ showed limited rescue of Lmo4 expression in the occipital cortex of KO;iz/hCOUP-TFI brains compared with COUP-TFI KO s. This suggests that COUP-TFI may specifically promote the development of somatosensory ( Lmo4 -negative) rather than of sensory/caudal areas in general ( Fig. 6d ). 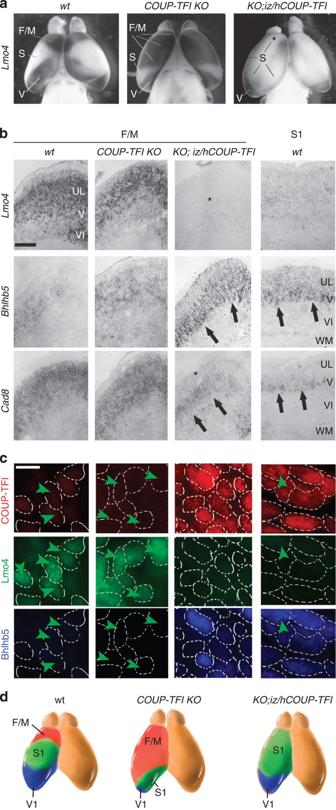Figure 6: F/M cortex acquires molecular somatosensory features after COUP-TFI overexpression. (a) Whole-mountin situhybridization showingLmo4expression inwt,COUP-TFI KOandKO;iz/hCOUP-TFIP0 brains.Lmo4is normally expressed in F/M and visual (V), but not in somatosensory (S) presumptive areas. InCOUP-TFI KOs, rostralLmo4expression is caudally expanded. Postmitotic overexpression of COUP-TFI (KO;iz/hCOUP-TFI) partially rescues caudalLmo4expression and downregulates its expression in S and F/M domains (asterisk). (b) Details of P0 F/M and prospective primary somatosensory (S1) cortical sections hybridized withLmo4,Bhlhb5andCad8riboprobes. Lmo4andCad8are strongly expressed inwtandCOUP-TFI KOF/M regions. InKO;iz/hCOUP-TFIbrains,Cad8is mainly restricted to layer V (black arrows) and downregulated in UL (asterisk), whereasLmo4is downregulated in all layers (asterisk). These expression profiles are reminiscent of those observed in S1 regions ofwtbrains.Bhlhb5is expressed at low levels in wt andCOUP-TFI KOF/M regions and re-expressed inKO;iz/hCOUP-TFIbrains in a pattern similar to the one found inwtS1 (black arrows). (c) Details of cortical neurons in F/M and S1 regions immunolabelled for COUP-TFI, Bhlhb5 and Lmo4. Note that low expression of COUP-TFI inwtand inCOUP-TFI KOrostral cortical neurons coincides with high Lmo4 and low Bhlhb5 expression levels, whereas high COUP-TFI expression inKO;iz/hCOUP-TFIand S1 areas correlates with low Lmo4 and high Bhlhb5 expression levels. Dashed lines designate the boundaries of labelled cell nuclei. (d) Schematic model of COUP-TFI-mediated areal identity specification in neocortex. Although F/M areas (red) are caudalized inCOUP-TFI KObrains, and S1 (green) and V1 (blue) areas are reduced and shifted to the occipital pole, ectopic expression ofhCOUP-TFIin frontal areas (KO;iz/hCOUP-TFIbrains) inhibits motor identity and promotes S1 expansion. This model is based on data obtained by molecular and connectivity analysis performed on the different genotypes. Scale bars, 1 mm (a), 40 μm (b), 20 μm (c). All panels are representative images of three independent experiments for each genotype. Figure 6: F/M cortex acquires molecular somatosensory features after COUP-TFI overexpression. ( a ) Whole-mount in situ hybridization showing Lmo4 expression in wt , COUP-TFI KO and KO;iz/hCOUP-TFI P0 brains. Lmo4 is normally expressed in F/M and visual (V), but not in somatosensory (S) presumptive areas. In COUP-TFI KOs , rostral Lmo4 expression is caudally expanded. Postmitotic overexpression of COUP-TFI ( KO;iz/hCOUP-TFI ) partially rescues caudal Lmo4 expression and downregulates its expression in S and F/M domains (asterisk). ( b ) Details of P0 F/M and prospective primary somatosensory (S1) cortical sections hybridized with Lmo4 , Bhlhb5 and Cad8 riboprobes . Lmo4 and Cad8 are strongly expressed in wt and COUP-TFI KO F/M regions. In KO;iz/hCOUP-TFI brains, Cad8 is mainly restricted to layer V (black arrows) and downregulated in UL (asterisk), whereas Lmo4 is downregulated in all layers (asterisk). These expression profiles are reminiscent of those observed in S1 regions of wt brains. Bhlhb5 is expressed at low levels in wt and COUP-TFI KO F/M regions and re-expressed in KO;iz/hCOUP-TFI brains in a pattern similar to the one found in wt S1 (black arrows). ( c ) Details of cortical neurons in F/M and S1 regions immunolabelled for COUP-TFI, Bhlhb5 and Lmo4. Note that low expression of COUP-TFI in wt and in COUP-TFI KO rostral cortical neurons coincides with high Lmo4 and low Bhlhb5 expression levels, whereas high COUP-TFI expression in KO;iz/hCOUP-TFI and S1 areas correlates with low Lmo4 and high Bhlhb5 expression levels. Dashed lines designate the boundaries of labelled cell nuclei. ( d ) Schematic model of COUP-TFI-mediated areal identity specification in neocortex. Although F/M areas (red) are caudalized in COUP-TFI KO brains, and S1 (green) and V1 (blue) areas are reduced and shifted to the occipital pole, ectopic expression of hCOUP-TFI in frontal areas ( KO;iz/hCOUP-TFI brains) inhibits motor identity and promotes S1 expansion. This model is based on data obtained by molecular and connectivity analysis performed on the different genotypes. Scale bars, 1 mm ( a ), 40 μm ( b ), 20 μm ( c ). All panels are representative images of three independent experiments for each genotype. Full size image Finally, to corroborate molecular analysis, we challenged the path of motor and sensory thalamocortical connectivity in control and KO;iz/hCOUP-TFI brains by inserting DiI in the motor and DiD in the somataosensory cortex ( Fig. 7a,b ). As expected, DiI retrogradely labelled the ventrolateral nucleus rostrally and the Po nucleus caudally, while DiD diffused exclusively to the VPM caudally in controls ( Fig. 7a,b ). Strikingly, no DiI retrograde labelling reached the rostral ventrolateral thalamic nucleus in KO;iz/hCOUP-TFI brains, whereas both DiI and DiD diffused to the VPM caudally, where their patterns partially overlapped ( Fig. 7b ). However, a few DiI-positive cells were still detected in the Po nucleus, implying that a minor part of the F/M areal connectivity was unaltered. 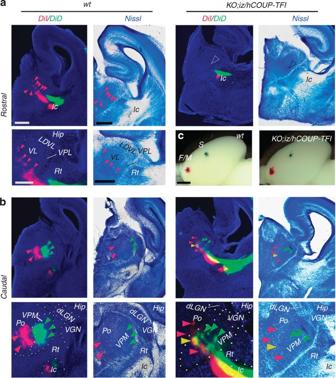Figure 7: Postmitotic COUP-TFI overexpression reroutes F/M areal connectivity. (a) Adjacent P0 brain coronal sections showing parietal cortex and rostral thalamus stained with DAPI (left panels of each genotype) and Nissl (right panels of each genotype). DiI and DiD crystals (red and green in fluorescent images, respectively) were inserted in the frontal and parietal cortices, respectively (see alsoc). Inwtbrains, DiI retrogradely labels cells of the ventrolateral nucleus (VL) (red arrowheads), whereas inKO;iz/hCOUP-TFIbrains, neither DiI or DiD label the VL (empty arrowhead). Panels under wt coronal sections represent higher magnifications of the regions labelled by DiI. Dotted lines in DAPI-stained sections depict the boundaries of thalamic nuclei. (b) Adjacent P0 brain coronal sections showing parietal cortex and mediocaudal thalamus stained with DAPI (left panels of each genotype) and Nissl (right panels of each genotype). Inwtbrains, DiI (inserted in the frontal cortex) retrogradely labelled cells of the Posterior nucleus (Po) (red arrowheads), whereas DiD (inserted in the parietal cortex) labels cells of the ventral posteromedial nucleus (VPM, green arrowheads). InKO;iz/hCOUP-TFIbrains, both DiI or DiD label the VPM, and their staining partially overlap (yellow arrowhead). Few DiI-labelled cells were also observed in the Po. Square panels under coronal sections represent higher magnifications of the regions labelled by lipophilic dyes. Dotted lines in DAPI-stained sections depict the boundaries of thalamic nuclei. (c) Images depicting the site of insertion of DiI (red) and DiD (blue) in the cerebral cortex of whole P0 brains. Hip, hippocampus; dLGN, dorsal lateral geniculate nucleus; Rt, reticular nucleus; VGN, ventral geniculate nucleus, VPL, ventral posterolateral nuclei; ic, internal capsule. Scale bars, 600 μm (coronal sections), and 300 μm (higher magnifications) (a,b), 1 mm (c). All panels of this figure are representative images of at least three independent experiments for each genotype. Figure 7: Postmitotic COUP-TFI overexpression reroutes F/M areal connectivity. ( a ) Adjacent P0 brain coronal sections showing parietal cortex and rostral thalamus stained with DAPI (left panels of each genotype) and Nissl (right panels of each genotype). DiI and DiD crystals (red and green in fluorescent images, respectively) were inserted in the frontal and parietal cortices, respectively (see also c ). In wt brains, DiI retrogradely labels cells of the ventrolateral nucleus (VL) (red arrowheads), whereas in KO;iz/hCOUP-TFI brains, neither DiI or DiD label the VL (empty arrowhead). Panels under wt coronal sections represent higher magnifications of the regions labelled by DiI. Dotted lines in DAPI-stained sections depict the boundaries of thalamic nuclei. ( b ) Adjacent P0 brain coronal sections showing parietal cortex and mediocaudal thalamus stained with DAPI (left panels of each genotype) and Nissl (right panels of each genotype). In wt brains, DiI (inserted in the frontal cortex) retrogradely labelled cells of the Posterior nucleus (Po) (red arrowheads), whereas DiD (inserted in the parietal cortex) labels cells of the ventral posteromedial nucleus (VPM, green arrowheads). In KO;iz/hCOUP-TFI brains, both DiI or DiD label the VPM, and their staining partially overlap (yellow arrowhead). Few DiI-labelled cells were also observed in the Po. Square panels under coronal sections represent higher magnifications of the regions labelled by lipophilic dyes. Dotted lines in DAPI-stained sections depict the boundaries of thalamic nuclei. ( c ) Images depicting the site of insertion of DiI (red) and DiD (blue) in the cerebral cortex of whole P0 brains. Hip, hippocampus; dLGN, dorsal lateral geniculate nucleus; Rt, reticular nucleus; VGN, ventral geniculate nucleus, VPL, ventral posterolateral nuclei; ic, internal capsule. Scale bars, 600 μm (coronal sections), and 300 μm (higher magnifications) ( a , b ), 1 mm ( c ). All panels of this figure are representative images of at least three independent experiments for each genotype. Full size image Taken together, these data suggest that ectopic expression of COUP-TFI in F/M cortex was sufficient to reroute rostral VPM thalamocortical innervation, and confirms that motor cortex of KO;iz/hCOUP-TFI brains acquires somatosensory-like properties. It is believed that positional information of areal identity is dictated by a combinatorial code of transcription factors expressed in gradients along the mediolateral and rostrocaudal coordinates of the developing cortex [6] , [9] , [46] . This transcriptional code shapes in progenitors a first rough areal map (protomap) [2] , which influences the following specification of newborn neurons. A second wave of transcription factors expressed postmitotically would then interpret the positional information initially coded in progenitor cells and impart areas their final properties [14] , [15] , [28] . This scenario is mainly based on mouse models in which several mitotically and postmitotically expressed genes were genetically manipulated, resulting ultimately in changes of the size and position of neocortical areas. As expected, alterations in expression levels of these patterning genes led to areal changes in accordance with their expression gradient [6] , [47] . However, the exact roles of mitotic and postmitotic gene gradients in the final specification of areal properties and how the primordial areal map is translated from progenitors to newborn neurons are still under debate. Are cortical neurons irreversibly committed to their final areal fate at the progenitor level? Do postmitotic patterning genes add new information and finally determine identities? Our study shows that a key regulator of neocortical arealization, such as COUP-TFI [44] , expressed in cortical progenitors and neurons in a caudolateral high to rostromedial low gradient, promotes sensory areal identity mainly in postmitotic cells. First, loss of postmitotic COUP-TFI function leads to a shift from sensory to motor identity in parietal neocortical neurons despite the presence of COUP-TFI expression in mitotic cells. Second, reintroducing COUP-TFI expression in COUP-TFI- null brains partly rescues the altered expression of areal markers and the incorrect positioning of thalamocortical connections. Third, ectopic COUP-TFI expression in rostral neurons, which normally lack this factor or express it at low levels, re-specify them to sensory identity. Thus, COUP-TFI expression in progenitors appears dispensable for sensory areal definition, whereas its activity in postmitotic cells appears to be necessary and sufficient to impart sensory identity to newly born neocortical neurons by controlling both sensory-specific gene expression and TCA topography. This does not exclude a fundamental role for Emx2 , which is still expressed in all COUP-TFI mutants analysed so far, and for other unknown mitotic patterning genes in sensory areal specification. However, our data show that the rostral expansion of sensory markers and connectivity observed in KO;iz/hCOUP-TFI is not dependent on Emx2 and/or mitotic COUP-TFI , which are not expressed in rostral progenitors. COUP-TFI postmitotic overexpression also shows an incomplete rescue of visual thalamocortical connections and a limited recovery of Lmo4 expression in the prospective visual cortex. These data lead to some interesting considerations on the postmitotic function of COUP-TFI in the cortex. On one hand, we have shown that overexpression of COUP-TFI in cortical neurons promotes somatosensory-specific features, such as downregulation of Lmo4 and thalamocortical VPM connectivity in motor and visual areas. This may argue for a prevalent role of COUP-TFI in the specification of somatosensory areas and correlates well with previous studies showing that genetic alterations in Emx2 expression, whose dorsoventral gradient in the caudal cortex is complementary to COUP-TFI, affect mainly the V1 size [48] , [49] . On the other hand, the incomplete rescue of normal TCA topography in KO;iz/hCOUP-TFI mice might be due to the absence of COUP-TFI expression in dorsal thalamic nuclei, as the Nex-Cre does not allow re-expression of COUP-TFI in the thalamus, and implies that reintroducing COUP-TFI only in the cortex and not in the thalamus fails to completely re-establish thalamocortical connectivity. Moreover, although cortical inactivation of COUP-TFI affects TCA topography (ref. 18 and this study), constitutive loss of COUP-TFI impairs TCA pathfinding as well (ref. 21 and our unpublished data), supporting independent roles of COUP-TFI in the cortex and in the thalamus during neocortical development (see also ref. 33 ). Thus, the remarkable rescue of sensory thalamo-cortical innervation after COUP-TFI cortical overexpression might be due to the restored specification of cortical SP neurons, which extend their axons towards the dorsal thalamic nuclei favouring correct TCA positioning in the neocortex [34] , [50] , [51] , [52] , [53] . Finally, we cannot exclude a direct control of COUP-TFI postmitotic gradient on molecular cues driving TCA pathfinding. Our data suggest that COUP-TFI is required in the regional specification of SP cells along the antero-posterior axis. As the SP is known to guide thalamic innervation into the cortex, the COUP-TFI gradient in these cells might guide thalamic axons to their proper target by controlling the expression of guidance molecules in an area-specific manner. However, it was previously shown that correct TCA topography needs molecular signals from both the SP and the CP [54] . If the action of COUP-TFI was just limited to the SP, we would observe only mild or no changes in the final TCA innervation of COUP-TFI KO s and KO;iz/hCOUP-TFI cortices. Thus, we propose that COUP-TFI may act in both SP and CP cells in guiding thalamic axons to their corresponding area. Further studies are needed to verify this hypothesis. Our study also shows that postmitotic COUP-TFI expression has an important role in neocortical lamination; however, we observed few differences in early-born (SP and layer VI) neuron specification and distribution between Emx- and NexCKO s, probably due to a role of mitotic COUP-TFI and of other mitotic patterning genes in these events. This is conceivable, as the first neuronal populations are born at a stage (E10.5) in which proliferating cells prevalently constitute embryonic cortices, and thus the influence of postmitotically active genes might be absent or less effective. Hence, alterations in the expression of mitotic patterning genes might impinge more significantly on early-born neuron specification. This supports an important role for mitotic patterning genes in area-specific commitment, as previously reported by the work on Emx2 , Sp8 and Pax6 (reviewed in refs 6 , 9 ). Accordingly, the COUP-TFI-mediated postmitotic to mitotic feedback, shown in our study, suggests that correct arealization asks for a dynamic fine-tuning of mitotic gene expression during corticogenesis. This feedback seems to act principally on Sp8 and mitotically expressed COUP-TFI during early corticogenesis and corroborates previous evidence demonstrating a reciprocal regulation between these two factors [40] . However, in our study, increased levels of Sp8 observed in Nex- and EmxCKO s cannot explain the massive expansion of motor areas observed in COUP-TFI mutants. Indeed, even if Sp8 promotes rostral areal specification, previous studies demonstrated that rostral Sp8 overexpression reduces rather than favour F/M areal identity [41] . In addition, the gradual increase in Sp8 expression from Nex- to EmxCKOs does not correlate with the severity of their areal phenotype, which is instead comparable between the mutants. Finally, loss and gain of postmitotic COUP-TFI function in the animal models analysed in this study starts around E11.5, that is, after the peak of action of rostralizing factors [42] , [55] . Thus, it is unlikely that late alterations in rostral patterning gene expression contribute to the observed areal impairments in COUP-TFI mutants. However, our data do not exclude that in normal conditions mitotic patterning genes regulate postmitotic COUP-TFI function by influencing its expression profile. Thus, they might indirectly define sensory areal boundaries by regulating COUP-TFI gradients. In summary, we propose that areal patterning genes in the germinative zone establish a co-ordinate system of positional information that needs to be corroborated in newborn neurons before being implemented. As postmitotic expression of COUP-TFI can act on sensory areal specification independently of COUP-TFI expression in progenitors, we hypothesize that postmitotically expressed genes not only reinforce positional information decided by the progenitors but also play key roles during areal identity specification. In support of this, we show that COUP-TFI postmitotic overexpression not only reverts a large number of features of the KO mutant areal phenotype but also reprogrammes neocortical neurons from motor to sensory identity (as shown by Lmo4 and Bhlhb5 respective expressions) in frontal regions. Notably, these data also indicate that areal patterning is a more plastic process than previously expected and invite a re-thinking of functional hierarchies between events taking place at progenitor and neuronal levels during neocortical arealization. Animals All mouse experiments were conducted according to national and international guidelines, and have been approved by the local ethics committee (CIEPAL NCE/2011-23). COUP-TFI fl/fl mice were either crossed to Emx1-Cre mice to inactivate COUP-TFI in progenitors ( COUP-TFI fl/fl EmxCre ) [18] or to NexCre mice [23] for COUP-TFI inactivation in postmitotic cells ( COUP-TFI fl/fl NexCre ). COUP-TFI KO mice were crossed to the NexCre and the CAGGS-lox-stop-lox-hCOUP-TFI [43] ( ind/hCOUP-TFI , conditionally expressing hCOUP-TFI under the control of β-actin promoter) mouse lines to reintroduce a human copy of COUP-TFI protein (hCOUP-TFI) in postmitotic mutant neocortical cells. These crosses produced several different genotypes in a Mendelian distribution. Among them, we analysed COUP-TFI+/+ NexCre- ind/hCOUP-TFI (iz/hCOUP-TFI ) and COUP-TFI−/− NexCre- ind/hCOUP-TFI ( KO;iz/hCOUP-TFI ) animals. Mouse lines were genotyped as previously described [16] , [18] , [23] , [43] . Midday of the day of the vaginal plug was considered as embryonic day 0.5 (E0.5). Control and mutant mice were predominantly bred in a C57BL6 background. Both male and female embryos and pups were used in this study. Post-mortem tissue collection Mice at P0 and P7 were intracardially perfused with paraformaldehyde (PFA) 4%. Embryonic and postnatal brain samples were fixed either for 2 h (for immunohistochemistry) or overnight (for in situ hybridization) at 4 °C in PFA 4%. Samples were then either embedded in optimal cutting temperature medium (JUNG) after being equilibrated to 30% sucrose and were cut on a Leica cryostat, or gradually dehydrated to 96% ethanol for whole-mount in situ hybridization. Samples to be used for floating immunohistochemistries, Nissl staining and lipophilic dyes- or cholera toxin-injected brains were embedded in 4% agarose after fixation and then cut on a Leica vibratome at 100 μm. No samples were excluded in this study, and for each experiment at least three animals from different litters were used. Immunohistochemistry and immunofluorescence Immunohistochemistries on cryosections were performed as previously described [16] , [18] . Briefly, for antigen unmasking, slides were boiled in sodium citrate 85 mM, pH 6.0. Slides were then blocked in 10% goat serum (newborn calf serum for 5-bromodeoxyuridine (BrdU) antibody), 0.1% Triton X-100 in PBS and incubated with primary antibodies overnight at 4 °C in 3% goat serum, 0.1% Triton X-100. For BrdU immunostaining, slides were first incubated in denaturation buffer (HCl 6.3%, 0.5% Triton in PBS) for 30 min at 37 °C and then in primary antibody as described above. The incubation with secondary antibodies was carried out for 2 h at room temperature. Ki-67 staining was amplified by the TSA Plus Cy3 System (PerkinElmer) following the manufacturer’s instructions. To detect the antigen in bright field, samples were incubated for 2 h in biotinylated anti-rabbit antibody (1:200; Vector), and then processed with the ABC kit (Vector) according to the manufacturer‘s instructions. Adding to the slides a Diaminobenzidine solution (Vector) revealed the expression of the antigen. Samples were then mounted in Aquatex (Merck). Samples treated for immunofluorescence were mounted with the following mounting solution: 80% glycerol, 2% N -propyl gallate, 1 μg ml −1 Hoechst (Invitrogen). To perform floating immunofluorescences, 100-μm-thick vibratome sections were first blocked overnight at 4 °C in 10% goat serum, 3% BSA and 0.1% Tween, and then incubated overnight with primary antibody at 4 °C in the same blocking solution. The sections were then incubated with the secondary antibody in the same conditions set for primary antibodies and mounted, the day after, as described above. The following primary antibodies were used: anti-BrdU (mouse, 1:100, Sigma), anti-c-Myc (rabbit, 1:250, Abcam; mouse 1:100, Santa Cruz), anti-COUP-TFI (rabbit, 1:1,000, manufactured and affinity purified on demand by Thermo-Fisher; because of the high homology between mouse and human COUP-TFI, the mouse COUP-TFI antibody can also recognize the human protein with high affinity), anti-Ctip2 (rat, 1:300, Abcam), anti-Cux1 (rabbit, 1:100, kind gift of A. Nepveu, Canada), anti-Fog2 (rabbit, 1:100, Santa Cruz), anti-Foxp2 (rabbit, 1:500, Abcam), anti-Ki67 (rabbit, 1:300, Spring), anti-5HT (rabbit, 1:500, Calbiochem), anti-Tbr1 (rabbit, 1:1,000, kind gift of R. Hevner, USA), anti-Tbr2 (rabbit, 1:1,000, Chemicon), anti-Tuj1 (mouse, 1:1,000, Covance), anti-Bhlhb5 (guinea pig, 1:35,000, kind gift of B. Novitch, USA) and anti-Lmo4 (rat, 1:1,000, kind gift of J. Visvader, Australia). The following secondary antibodies were used: anti-Rabbit FC 488, 594; anti-Rat FC 488, 594, 633; anti-Mouse FC 488, 594; anti-Guinea Pig FC 594 (1:300, Life Technologies). Each experiment was repeated at least three times. In situ hybridization For both in situ hybridization and whole mount in situ hybridization, please refer to the previously described protocols [18] , [56] . Briefly, for whole-mount in situs , brains stored in ethanol 96% were rehydrated and treated with a 0.5% hydrogen peroxide solution from 45 to 60 min depending on their age. Brains were then treated with 10 μg ml −1 PK (Roche) (30 to 45 min depending on their age) and post-fixed 15 min in 4% PFA/ 0.1% Tween-20 (Sigma)/0.1% glutaraldehyde (Sigma). Brains were then hybridized overnight at 70 °C to digoxigenin-labelled riboprobes in the following solution: 50% formamide, 1.3 × SSC, 5 mM EDTA, 50 μg ml −1 Yeast t-RNA (Invitrogen), 2% Tween, 0.5% CHAPS (Sigma). All washes from one step to the other were performed in PBS1/0.1% Tween-20. The day after, brains were washed twice for 1 h in hybridization solution and then equilibrated in TST (0.5 M NaCL, 10 mM Tris, pH 7.5, 0.1% Tween 20) to remove aspecifically hybridized riboprobes by RNAse A treatment (10 μg ml −1 ). Finally, the samples were equilibrated in MABT (100 mM maleate, 150 mM NaCl, 175 mM NaOH, 0.1% Tween 20, pH 7.5) to detect hybridized riboprobes by the use of an anti-DIG antibody (1:2,000, Roche) overnight at 4 °C. Detection of the antibody was performed by NBT/BCIP solution (Roche) at room temperature. In situ hybridizations on cryostat-cut brain sections were performed as follows. Defrosted and dried brain sections were treated with RIPA buffer (150 mM NaCl, 1% NP-40, 0.5% Na deoxycholate, 0.1% SDS, 1 mM EDTA, 50 mM Tris, pH 8.0) twice for 10 min and then postfixed 15 min in 4% PFA. Pre-hybridization and hybridization of the sections with riboprobes were performed at 70 °C in the following solution: 50% formamide, 5 × SSC, 5 × Denhardts solution (Invitrogen), 500 μg ml −1 Salmon Sperm DNA (Ambion) 250 μg ml −1 Yeast t-RNA. The day after, slides were washed twice for 1 h at 70 °C in the following solution: 50% formamide, 2 × SSC, 0.1% Tween 20. Then, the samples were equilibrated in MABT solution and blocked in MABT/10% sheep serum to detect the hybridized riboprobes by anti-DIG antibody (see above). Finally, sections were washed several times in MABT, equilibrated in B3 buffer (100 mM Tris, pH 9.5, 50 mM MgCl2, 100 mM NaCl, 0.1% Tween-20) and the antibody was detected incubating the slices in NBT/BCIP solution (see above). The riboprobes were synthesized by the use of DIG RNA labelling kit (Roche) following manufacturer’s instructions. Nissl staining For Nissl staining, 100-μm-thick sections were mounted on slides and left to dry for 15 min. The slides were briefly washed in MilliQ water and then immersed 5 min in the following staining solution: 0.025% thionine acetate (Sigma, T2029-5G), 0.025% Cresyl violet acetate (Sigma, T2029-5G), 100 mM sodium acetate, 8 mM acetic acid. Slides were then washed in ethanol 80%/acetic acid 0.05% for a variable time in function of the rate of clarification. Slides were finally dehydrated by two brief washes in ethanol 100% and finally two 5-min-long washes in xylene. Coverslips were mounted on slides by the use of Eukitt mounting medium (KO Kinder GmbH D-79110) paying attention to not let the slides dry before mounting. TCA tracing We used two independent approaches for tracing TCAs. The first one comprises injections of the CTB-conjugated fluorophores (Invitrogen, 488 nm C34775 and 555 nm C34776) in live animals. P4 pups were anaesthetized on ice and immobilized on a Digital Lab Standard Stereotaxic Instrument (Stoelting 51900). The skin was opened at the dorsal base of the skull to visualize the lambda ( λ ) point at the junction between parietal and occipital bones; once the needle loaded on the Nanoinjector (Nanoject II Auto-Nanoliter Injector, Drummond Scientific Company 3-000-204) was positioned in the centre of the λ , the x , y , z parameters were set to zero. The skull was then perforated with a glass needle to the desired position and 6 × 9.2 nl pulses of CTB were injected. Precise coordinates were registered during injections; however, variations in size of P4 pups and differences in the tension of the immobilized skull asked for regular re-adaption of the injections site during each experiment. Pups were left for 15 min on a warming plate at +37 °C for awakening and then given back to their mothers. Pups injected were killed at P7 by PFA perfusion and brains were subsequently fixed on. In the second approach, lipophilic crystals were placed into post-mortem P0 brains. After 2 h fixation in 4% PFA, crystals of DiI’ (DiIC18(3); Molecular Probes) and DiD’ (DiIC18(5); Molecular Probes) were inserted into defined brain regions. After 2 weeks in 2% PFA at 37 °C to allow lipophilic dyes diffusion, brains (three for controls and three for each mutant) were vibratome cut to obtain 100-μm-thick slices, which were mounted as described above (see ‘Immunohistochemistry and immunofluorescence’ section). Three controls and three mutant brains were processed and analysed for each tracing experiment described in the text. RNA extraction and complementary DNA synthesis RNA for microarray and reverse transcriptase–PCRs (RT–PCRs) was obtained from E12.5 and E15.5 neocortices (at least three biological samples for each genotype), and was extracted using the RNeasy Mini kit (Qiagen) following manufacturer’s instructions. cDNA was synthesized starting from 1 μg of total RNA using Superscript III First-Strand Synthesis System for RT–PCR (Invitrogen) following manufacturer’s instructions. Meninges were carefully removed from the samples before instant freezing in liquid nitrogen. Real-time PCR RT–PCRs on cDNA was performed using FAST SYBR Green Master Mix (Applied Biosystems) according to manufacturer’s instructions. Samples were run on a LigthCycler II 480 (Roche) and the following primers were used: GADPH FW: 5′-GTATGACTGCACTCACGGCAAA-3′; GADPH rev: 5′-TTCCCATTCTCGGCCTTG-3′; COUP-TFI FW: 5′-AGCTGCCTCAAAGCCATCGTG-3′; COUP-TFI rev: 5′-AGTTGCTCGATGACAGAGGAG-3′; Emx2 FW: 5′-TACCGATATCTGGGTCATCGC-3′; Emx2 rev: 5′-GGCGGTTCGAATCCGCTTTG-3′; Pax6 FW: 5′-TAGCGAAAAGCAACAGATG-3′; Pax6 rev: 5′-TCTATTTCTTTGCAGCTTCC-3′; Sp8 FW: 5′-TGACCGAAACATCAGGAAATGG-3′; Sp8 rev: 5′-CTATGCTCAGTTCTCCCGAGC-3′. Microarray implementation and analysis of data cDNA was generated from 200 ng of total RNA (from at least three brains for each genotype) using the WT Expression Kit (Ambion), according to manufacturer’s instructions. After fragmentation, cDNA was end-labelled using the GeneChip WT Terminal Labelling Kit (Affymetrix). Labelled DNA targets were hybridized to the Affymetrix GeneChip Mouse Gene 1.0 ST Array at 45 °C for 17 h, according to the manufacturer’s recommendation. Hybridized arrays were washed and stained on a GeneChip Fluidics Station 450 and scanned on a GeneChip Scanner 3000 7G (Affymetrix). Gene expression levels were summarized using Gene Level-RMA sketch method in the Expression Console software (Affymetrix). Normalized data were then analysed with the oneChannelGUI package from Bioconductor [57] , using the Benjamini & Hochberg (BH) adjust method. Microarray data (.matrix and.cel files) stored on Mediante, a web-based microarray data manager [58] , [59] , have been deposited at the Gene Expression Omnibus with accession number GSE52395. Gene set analysis Rostrocaudal gene sets were updated and modified from Elsen et al. [38] , by using the same sources and approaches described there. Briefly, genes that exhibit zonal rostrocaudal expression gradients were grouped according to predominant expression in the CP, SP, IZ, intermediate progenitors mainly in the subventricular zone, or VZ. Changes in the expression levels of each gene, represented as log 2 of the fold change (log 2 FC), were determined by microarray. Gene sets were summarized by determining the mean change in log 2 FC and the s.e.m. for all genes in the set. Statistical analysis All counting made on images were performed with ImageJ, setting the threshold for single channels and using the analyse particle algorithm after applying the watershed algorithm to separate close objects. The same thresholds used for single-channel counting were also employed for the co-localization analysis, which was performed using the object-based method of the JACoP plugin [60] . Every counting was performed on at least three samples ( n =3) for each genotype. The mean value for each group was calculated using the averages from three adjacent sections of each sample. To evaluate statistical significance, we used two-tailed t -test analysis when comparing two different groups and single factor ANOVA (analysis of variance) when comparing three groups. The post-hoc analysis was performed again by two-tailed t -test. The statistical error was expressed as s.e.m. Data were considered significant when P ≤0.05. Image acquisition Whole-brain images were acquired with a Leica Z16 APOA macroscope. In situ hybridizations, immunohistochemistries, Nissl stainings and immunofluorescences were acquired with either a LEICA DM6000 microscope equipped with LEICA DFC 310 FX camera or with a ZEISS Imager.Z1 microscope equipped with AXIOCAM MRm camera. Details of thick sections were taken with a confocal ZEISS 780 microscope. How to cite this article: Alfano, C. et al. Postmitotic control of sensory area specification during neocortical development. Nat. Commun. 5:5632 doi: 10.1038/ncomms6632 (2014). Accession codes: Microarray data have been deposited at the Gene Expression Omnibus (GEO) with accession number GSE52395 .